Simple push coating of polymer thin-film transistors A primary step in solution-based organic semiconductor processing is the formation of a thin liquid–solution layer on a substrate surface, produced either by spin coating, casting, dipping or painting (that is, printing) [1] , [2] , [3] , [4] , [5] , [6] , [7] . The thickness of the solution layer typically ranges between 0.1–100 μm, from which thin solid films 10–1,000 nm in thickness are obtained by the subsequent evaporation of solvent. However, the fluidic nature of solutions is contradictory to liquid-layer formation on highly hydrophobic surfaces because solutions should exhibit rapid shrinkage to form a thick hemispherical droplet. The feature causes a serious dilemma in the solution processes, as the use of such surfaces is indispensable for improving device characteristics [8] , [9] , [10] , [11] , [12] , [13] . Spin coating is widely utilized to produce a temporary thin solution layer, although considerable material loss is inevitable in the initial spinning process [14] . It is also difficult to use high boiling point (b.p.) solvents owing to the temporary nature of the film formation, although their use is effective for achieving highly crystalline films [15] . Contact cast methods, which include blade coating or slot-die coating in a broad sense, are utilized to confine the solution to a thin narrow space using a contact plane such as a metal bar, or a glass or plastic plate [1] , [2] , [4] , [6] . Using these techniques, the substrate surfaces can be wetted by capillary force, while solvent evaporation occurs only at the solution–air interface located at the edges of the contact plane. Such a spatial difference between solidification and solvent evaporation causes non-uniformity and material loss. In contrast, a poly(dimethylsiloxane) (PDMS) stamp is utilized in printing techniques to transfer semiconductor films to substrates by virtue of the semiwet nature of PDMS [16] , [17] , [18] , [19] . Nonetheless, film transfer onto hydrophobic surfaces remains difficult because the films detach easily from the low-surface-energy surface when the drying stamp is peeled off. Considerable material loss is also inevitable in the initial inking process on top of the stamps. Here we present an extremely simple ‘push coating’ technique that combines the contact casting and transfer printing where the PDMS elastomer is utilized both as the pressing contact plate and as the solvent extraction media from the solution. A solution layer is formed by the capillarity-induced wetting of the surface by a conformal contact with the PDMS-based trilayer stamp. Then the semiconductor films are grown through the solvent sorption to the stamp. We show that the subsequent solvent retention in the stamp allows the stamp to be peeled perfectly from the semiconducting polymer film fabricated even on highly hydrophobic surfaces and after the long stamping time required for film growth. Although the sorptive and retentive nature to a variety of organic solvents has been regarded as a drawback of PDMS [20] , [21] , the behaviour is utilized as the fundamental basis in this technique. We have applied the technique to a typical semiconducting polymer, poly(3-hexylthiophene) (P3HT), and clearly demonstrated the improved crystallinity and enhanced mobility in the thin-film transistors (TFTs). We suggest that the technique is both useful and readily applicable to thin-film processing of a wide range of materials. Film processing by push coating The first step of the push-coating technique is to produce a thin semiconductor solution layer on a substrate surface by compressing a microlitre solution droplet with a viscoelastic PDMS-based stamp, as presented in Fig. 1a . We designed a PDMS/fluorocarbon polymer/PDMS trilayer stamp in which the PDMS layers work as both-sided surface-contact layers and the fluorocarbon polymer works as a blocking layer against solvent diffusion [22] ( Fig. 1b ). The use of the trilayer structure is effective in promoting solvent retention within the stamp as well as in minimizing stamp deformation against solvent sorption. More importantly, it was found that the lasting solvent retention in the stamp allows perfect peeling of the stamp from the semiconducting polymer films even after a very long stamping duration for the film growth. 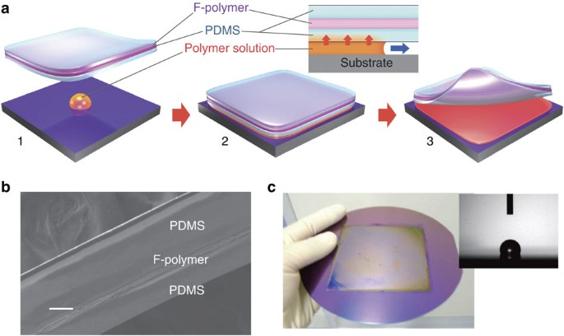Figure 1: Push coating of semiconducting polymer films. (a) Schematic of the process. A droplet of the semiconductor solution is first placed on a substrate (step 1), and the solution is compressed by the PDMS/fluorocarbon (F)-polymer/PDMS trilayer stamp to form a solution layer at the interface. Subsequent solvent sorption and retention by the stamp allows gradual growth of the semiconductor film (step 2). The stamp is then peeled off, leaving a whole film on the substrate (step 3). (b) Scanning electron microscope image of the trilayer stamp. (c) A polymer film on a 6-inch Si wafer with a highly hydrophobic surface treated with 1H,1H,2H,2H-perfluorodecyltriethoxysilane; the water contact angle (right) is larger than 110°. The scale bar inbrepresents 100 μm. Figure 1: Push coating of semiconducting polymer films. ( a ) Schematic of the process. A droplet of the semiconductor solution is first placed on a substrate (step 1), and the solution is compressed by the PDMS/fluorocarbon (F)-polymer/PDMS trilayer stamp to form a solution layer at the interface. Subsequent solvent sorption and retention by the stamp allows gradual growth of the semiconductor film (step 2). The stamp is then peeled off, leaving a whole film on the substrate (step 3). ( b ) Scanning electron microscope image of the trilayer stamp. ( c ) A polymer film on a 6-inch Si wafer with a highly hydrophobic surface treated with 1H,1H,2H,2H-perfluorodecyltriethoxysilane; the water contact angle (right) is larger than 110°. The scale bar in b represents 100 μm. Full size image A photograph of one obtained film is presented in Fig. 1c . To form a film with an area of 85 × 85 mm 2 , we used a droplet of P3HT in 0.1 wt% 1,2,4-trichlorobenzene (TCB) solution with a volume of about 350 μl. The droplet was placed at around the centre of the substrate, and then the stamp, supported by a 0.6-mm-thick glass plate, was adhered uniformly to the highly hydrophobic substrate surface. The solution layer spread across the entire stamp–substrate interface. The stamp was pressed with a moderate pressure of ~135 Pa (using a 100 g weight) and was annealed for 5–20 min at 25–150 °C, during which time the solvent was slowly absorbed by the stamp. Then the stamp was peeled off, leaving a whole polymer film adhered to the substrate. All the above-mentioned processes were conducted in air. Finally, all the films were annealed at 150 °C for 15 min and 165 °C for 5 min in a N 2 -filled glove box. Thickness of the films ranges between 10–1,000 nm, which can be controlled by selecting the concentration and volume of the semiconductor solution. The facile peeling capability of the stamp is evidently associated with the sorptive and retentive nature of PDMS to a variety of organic solvents [20] . The stamp was slightly swollen when peeled off as a result of solvent retention. We measured the total weight variation of the PDMS stamp after it had been soaked in chloroform or TCB and as it dried after being drawn from the solvent; the results are shown in Fig. 2a . We found that the weight variations (Δ M ) in all four cases are well reproduced by a simple exponential function: Δ M = A exp(− t / t 0 ). The absorption and desorption time ( t 0 ) of TCB by the PDMS is estimated to be about 1,000 and 40,000 s, respectively. This indicates that the stamp–film interface should be kept semiwet for a long period of time, while the film–substrate interface should be dried quickly. In Fig. 2b , the surface coverage ratio of the P3HT films on the substrate, when the stamp is peeled off, is plotted as a function of the stamping time. The peeling capability, that is, the ability to leave a whole film on the substrate, lasts even on highly hydrophobic surfaces and after an infinitely long stamp time. This feature can be attributed to the fact that the adhesion force between solid materials is considerably reduced in the presence of fluid molecules [23] . These results demonstrate that the push-coating technique enables us to form completely uniform semiconductor films on a highly hydrophobic surface through the use of a high b.p. solvent, which is in stark contrast to the case of spin coating that only affords films showing a fairly low coverage ( Supplementary Fig. S1 ). In addition, push coating uses all the available material for the film formation; the feature should be an enormous advantage in realizing material cost reductions in the electronic device productions. We also consider that the technique could be easily scaled up to cover a larger area of more than 10–100 times, as it takes about a minute for the stamp to fully absorb the solvent. 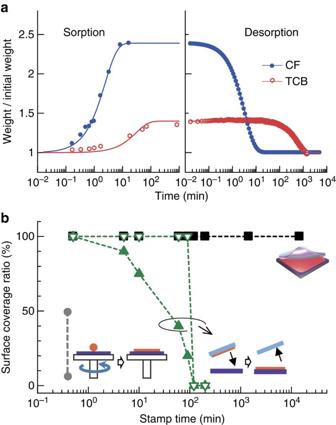Figure 2: Solvent sorption properties and peeling capability of the trilayer stamp. (a) Total weight variation (ΔM) of the dry stamp after soaking in chloroform (CF) or TCB (left), shown as filled and open circles, respectively, and that of the fully soaked stamp drying after being drawn from the solvent (right). The solid curves are a fit to the equation ΔM=A exp(−t/t0). (b) The stamp-time dependence of the surface coverage ratio (ratio of surface area covered by the films to the whole surface area) for the push-coated semiconducting polymer films both on a hydrophobic or hydrophilic substrate (both with filled squares) and for the transfer-printed films on a hydrophobic (filled triangles) and hydrophilic (open triangles) substrates. The surface coverage ratio for the spin-coated films is also shown by filled circles. Figure 2: Solvent sorption properties and peeling capability of the trilayer stamp. ( a ) Total weight variation (Δ M ) of the dry stamp after soaking in chloroform (CF) or TCB (left), shown as filled and open circles, respectively, and that of the fully soaked stamp drying after being drawn from the solvent (right). The solid curves are a fit to the equation Δ M =A exp(− t / t 0 ). ( b ) The stamp-time dependence of the surface coverage ratio (ratio of surface area covered by the films to the whole surface area) for the push-coated semiconducting polymer films both on a hydrophobic or hydrophilic substrate (both with filled squares) and for the transfer-printed films on a hydrophobic (filled triangles) and hydrophilic (open triangles) substrates. The surface coverage ratio for the spin-coated films is also shown by filled circles. Full size image Fine film patterning Push coating not only provides plane films but also allows us to use a variety of fine patterning processes because the films can in principle be manufactured on any flat surface. A simple example of the push-coating pattering process is illustrated in Fig. 3a . We used two sets of PDMS sheets; one is used as a substrate for the initial push coating as well as a blanket for subsequent transfer printing, and another as a stamp for the push coating. A plane semiconducting polymer layer is first fabricated on the former PDMS substrate by push coating with use of the latter PDMS stamp. The stamp is preheated at 65 °C so that the stamp has higher sorptive nature than the substrate [24] . By the preheat treatment, a whole semiconductor film remains on the PDMS substrate after the PDMS stamp is peeled off. The film on the PDMS substrate is then pressed onto a pattern-moulded glass plate that has a higher surface energy than the substrate surface, and the unnecessary parts of the film are removed to obtain the patterned film. Finally, the patterned films were transferred from the PDMS substrate (or blanket) to a target highly hydrophobic substrate treated with trichloro(1H,1H,2H,2H-perfluorooctyl)silane (FOTS-8). A micrograph of patterned semiconducting polymer films with 200 p.p.i. resolution is presented for P3HT, poly(3,3′″-didodecyl quarter thiophene) (PQT-12) [13] and poly(2,5-bis(3-hexadecyl thiophen-2-yl)thieno (3,2- b )thiophene) (PBTTT) [25] in Fig. 3b ; note that material loss is only limited to the unnecessary parts of the film in the process. 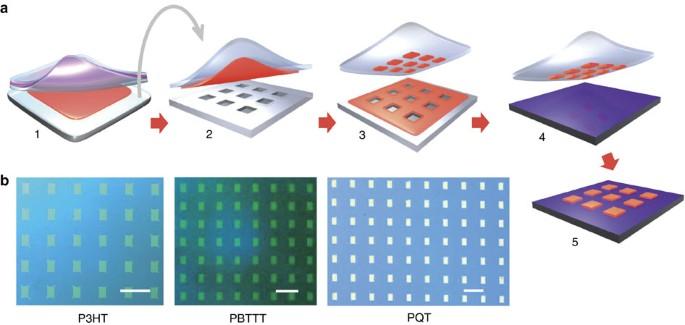Figure 3: Patterning process for push-coated flat films. (a) Schematic of the process. Negative image patterning by a moulded glass plate for the push-coated semiconducting polymer films on a PDMS stamp (steps 1 and 2), and transfer printing of the patterned films from the stamp to a substrate (steps 3 and 4). (b) Micrographs of the patterned films with a 200 p.p.i. resolution on highly hydrophobic SiO2substrates treated with trichloro(1H,1H,2H,2H-perfluorooctyl)silane. The following three kinds of semiconducting polymers are used for the demonstration; P3HT, PBTTT and PQT-12. The scale bars inbrepresent 100 μm. Figure 3: Patterning process for push-coated flat films. ( a ) Schematic of the process. Negative image patterning by a moulded glass plate for the push-coated semiconducting polymer films on a PDMS stamp (steps 1 and 2), and transfer printing of the patterned films from the stamp to a substrate (steps 3 and 4). ( b ) Micrographs of the patterned films with a 200 p.p.i. resolution on highly hydrophobic SiO 2 substrates treated with trichloro(1H,1H,2H,2H-perfluorooctyl)silane. The following three kinds of semiconducting polymers are used for the demonstration; P3HT, PBTTT and PQT-12. The scale bars in b represent 100 μm. Full size image Thin-film characteristics Push coating has a wide range of controllable nature in terms of film processing that allows the gradual growth of highly crystalline semiconducting polymer films. Figures 4 and 5 examine the crystallinity of push-coated films grown under various processing conditions (that is, different solvents and temperatures; see Methods). We found that the processing duration is not important, if it is longer than the time for solvent sorption. The atomic force microscope images for the film surface morphology are shown in Fig. 4a . The film grown at room temperature presents a fibril-type surface morphology in the push-coated film, which is in contrast to the fairly flat surface morphology in the spin-coated film. The feature should be associated with the film growth contacted with PDMS stamps. We also found that the push-coated film surfaces have a higher flatness when processed at a higher temperature, where the fibril-type morphology disappears. The feature should indicate the improved crystallinity on the film surface. Actually, out-of-plane Bragg diffraction up to third order was observed in the push-coated films, while second- or third-order diffraction was weak in the spin-coated films ( Fig. 4b and Supplementary Fig. S2 ). By the results, we conclude that a higher crystallinity should be achieved in the push-coated films. 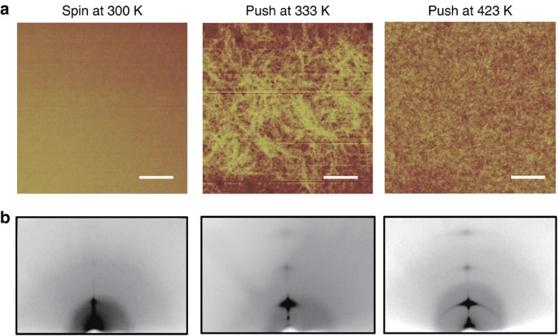Figure 4: Surface morphology and out-of-plane diffraction. (a) Atomic force microscope images and (b) X-ray oscillation photographs of the P3HT films processed by spin coating at 300 K, and push coating at 333 and 423 K, respectively (all with TCB and OTS-18-treated SiO2surface). The scale bars inarepresent 2 μm. Figure 4: Surface morphology and out-of-plane diffraction. ( a ) Atomic force microscope images and ( b ) X-ray oscillation photographs of the P3HT films processed by spin coating at 300 K, and push coating at 333 and 423 K, respectively (all with TCB and OTS-18-treated SiO 2 surface). The scale bars in a represent 2 μm. 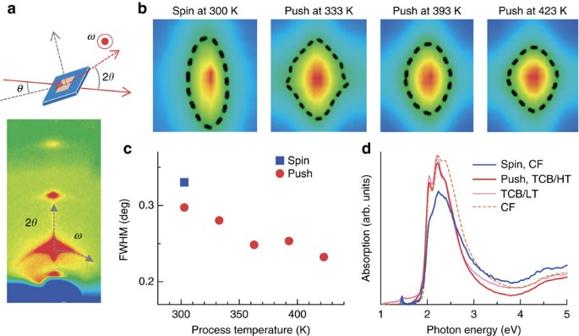Figure 5: Crystalline nature of push-coated P3HT films. (a) An oscillation photograph (Δθ=5°) of the push-coated film. (b) Peak profiles of the out-of-plane (100) X-ray diffraction for the films processed by spin coating at 300 K, and push coating at 333, 393 and 423 K, all of which are fabricated with TCB solution and OTS-18-treated SiO2surfaces. The dashed curves exhibit the contours at half maxima of the Bragg peak intensity, respectively. (c) Process-temperature dependence of the (100) diffraction peak width (full width at half maximum) for the spin- and push-coated films. (d) Ultraviolet/visible absorption spectra of the films fabricated by spin coating with the chloroform (CF) solution, and by push coating with TCB solution at 423 K (HT) or 333 K (LT) or with CF solution at 300 K. Full size image Figure 5: Crystalline nature of push-coated P3HT films. ( a ) An oscillation photograph (Δ θ =5°) of the push-coated film. ( b ) Peak profiles of the out-of-plane (100) X-ray diffraction for the films processed by spin coating at 300 K, and push coating at 333, 393 and 423 K, all of which are fabricated with TCB solution and OTS-18-treated SiO 2 surfaces. The dashed curves exhibit the contours at half maxima of the Bragg peak intensity, respectively. ( c ) Process-temperature dependence of the (100) diffraction peak width (full width at half maximum) for the spin- and push-coated films. ( d ) Ultraviolet/visible absorption spectra of the films fabricated by spin coating with the chloroform (CF) solution, and by push coating with TCB solution at 423 K (HT) or 333 K (LT) or with CF solution at 300 K. Full size image Figure 5b presents contour curves of (100) diffraction peaks for films processed at various temperatures. We found that the width along 2 θ for the push-coated films is smaller than that for the spin-coated film, and it decreases with increasing processing temperature ( Fig. 5c ). In contrast, the width along ω remains almost constant (also see Supplementary Fig. S3 ). The widths along 2 θ and ω are almost same in the film processed at 423 K, indicating the homogeneous nature of the d spacing. In addition, the diffraction peak angle is slightly higher in the push-coated films than that in the spin-coated films. All the results indicate that the narrower peak width of the films processed at high temperatures can be ascribed to the homogeneous d spacing (=1.64 nm), while the spin-coated films are composed of grains with a distributed d spacing (1.64–1.69 nm). It means that the higher process temperature allows film growth with a higher crystallinity. As all the films are annealed at a higher temperature after the process, this implies that the control of film growth condition is more important than the post-annealing. In the ultraviolet-visible absorption spectra, the push-coated films also present discriminated side-band features more clearly than the spin-coated films, providing consistent evidence of the higher crystallinity in the push-coated films [16] , [26] ( Fig. 5d ). Thin-film transistors The higher crystallinity of the push-coated films affords high carrier mobility. We fabricated bottom-gate, bottom-contact P3HT TFTs using the push-coated and spin-coated polymer films obtained with various solvent and surface treatment combinations (Methods). All the devices present typical TFT characteristics ( Fig. 6 ), and we estimated the field-effect mobility μ and threshold voltage V T in the saturation regime ( V D =−80 V). The μ for push-coated films with TCB solution on an trichloro(octadecyl)silane (OTS-18)-treated surface was 0.34 cm 2 V −1 s −1 . For films with chloroform solution on a 1,1,1,3,3,3-hexamethyldisilazane-treated surface, push coating gave a μ of 0.12 cm 2 V −1 s −1 , while spin coating produces a μ of 0.047 cm 2 V −1 s −1 . The highest push-coated P3HT TFT mobility was 0.47 cm 2 V −1 s −1 , which is ten times higher than that of the TFT fabricated by spin coating. 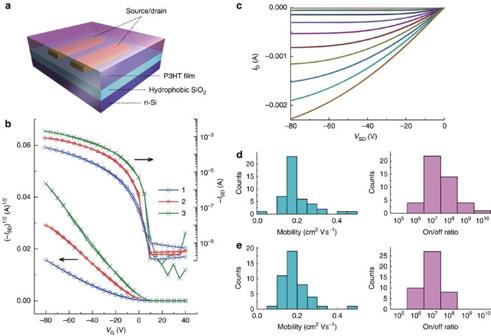Figure 6: Characteristics of TFTs based on push-coated P3HT films. (a) Schematic of the bottom-gate, bottom-contact TFT device structure. (b) Transfer characteristics (VSD=−80 V) of the device processed by 1: spin coating with chloroform (CF) solution on the 1,1,1,3,3,3-hexamethyldisilazane (HMDS) substrate, 2: push coating with CF solution on the HMDS substrate and 3: push coating with 1,2,4-TCB solution on the OTS-18 substrate (all at 333 K). (c) Typical output characteristics of the device. (d) Distribution of the mobility and on/off current ratio for devices processed by push coating with TCB solution at 333 K, and (e) at 423 K; both distributions are results from 45 transistors. Figure 6: Characteristics of TFTs based on push-coated P3HT films. ( a ) Schematic of the bottom-gate, bottom-contact TFT device structure. ( b ) Transfer characteristics ( V SD =−80 V) of the device processed by 1: spin coating with chloroform (CF) solution on the 1,1,1,3,3,3-hexamethyldisilazane (HMDS) substrate, 2: push coating with CF solution on the HMDS substrate and 3: push coating with 1,2,4-TCB solution on the OTS-18 substrate (all at 333 K). ( c ) Typical output characteristics of the device. ( d ) Distribution of the mobility and on/off current ratio for devices processed by push coating with TCB solution at 333 K, and ( e ) at 423 K; both distributions are results from 45 transistors. Full size image According to the previous reports, the μ values of P3HT are ranged between 0.01–0.4 cm 2 V −1 s −1 ( [7] , [16] , [26] , [27] , [28] ), and are affected not only by the film fabrication process but also by the material properties, such as the molecular weight or the regio-regularity. Although our source material is commercial and quite conventional one, the observed field-effect mobility is one of the highest for the P3HT. We conclude that the improvement can be clearly ascribed to the greater crystallinity of the push-coated films. We suggest that the push coating should be quite useful and as easily applicable in fabricating uniform thin films as spin coating. In contrast to general wet processes, including spin coating, the push coating has the following unique advantages: first, push coating is applicable to any substrate–solvent combination, including high b.p. solvents, and it is also not necessary to use any additional surfactants or mixed solvents for controlling the wettability on hydrophobic surfaces. Second, only a small amount of solution is necessary in push coating, and third, the process time, temperature, film thickness and coating area can be predefined. In conclusion, we have developed a very simple push-coating technique that is advantageous for low-cost production of high-performance, uniform and wide-area semiconducting polymer films on highly hydrophobic surfaces. The technique uses a tiny volume of a semiconducting polymer solution that is compressed by a PDMS-based trilayer stamp to form a thin solution layer confined between the stamp and the substrate. The unique nature of the process means that the semiwet nature at the stamp–film interface is preserved for a long period of time owing to the sorptive and retentive nature of the stamp to the solvents; this feature enables the stamp to be peeled perfectly from the films fabricated on any low-surface-energy substrates. We also demonstrated that the push coating on hydrophobic PDMS substrate can be followed by a simple fine pattering and transfer printing process. Application of P3HT as the semiconducting polymer clearly demonstrates improved crystallinity with homogenous d spacing and an enhanced field-effect mobility of the fabricated films. The technique should be applicable to thin-film processing of a wide range of materials, and we believe that the unique advantages of push coating will constitute a major step towards the low-cost production of flexible electronics products. Stamp fabrication We used a commercially available silicone that includes a hardening agent, KE106 (Shin-Etsu Chemical Co., Ltd.), to fabricate the PDMS elastomer, and SIFEL2610 (Shin-Etsu Chemical Co., Ltd.) for the fluorocarbon polymer elastomer that has similar mechanical characteristics with the PDMS. Each material was stirred and bubbles were removed with a vacuum pump (base pressure of 133 Pa). The stirred material was then poured onto a silica plate and sandwiched by another silica plate causing the silicone to spread between the plates. To form a large-size stamp or blanket, we used a printing device (PA 400s, Nanometric Technology Inc.) in order to ensure a parallel gap between the large-size silica plates, which was filled with silicone. Each silicone was hardened by a heat treatment in an oven or on a hot plate (at 150 °C for 30 min for the PDMS and at 150 °C for 60 min for the fluorocarbon polymer). After solidification, these elastomers were peeled from the silica plates and stacked with each other to form the trilayer stamp. For the facile peeling, we used silica plates whose surfaces were modified with 1H,1H,2H,2H-perfluorodecyltriethoxysilane (FAS-17). Finally, the stamp was cut into the desired shape. Photograph of a 4-inch-size trilayer stamp is presented in Fig. 7 . The typical thickness of fluorocarbon polymer layer is 50 μm, while that of the PDMS layer is ranging between 100–200 μm. The PDMS surface has superior flatness with a root-mean-square roughness of 1.20–1.36 nm. The fluorocarbon polymer layer we used has good adhesion properties with the PDMS layer, and it is difficult to be peeled from each other. The water contact angle of the stamp surface was 91°. In order to reduce the residual contamination in the stamp, we cleaned the stamp by acetone just before the use. We found that the stamp could be cured by solvent desorption and is reusable for at least more than 10 times. 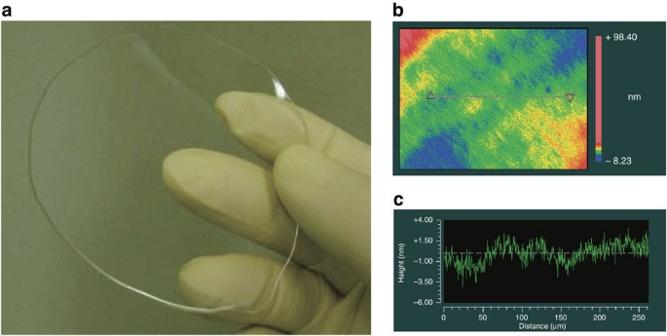Figure 7: Appearance of a trilayer stamp. (a) Photograph of a trilayer stamp. (b) A microscope image and (c) surface profile of the stamp monitored by a phase measurement with an interface microscope. The stamp surface has a high flatness because of the flatness of the glass plate. Figure 7: Appearance of a trilayer stamp. ( a ) Photograph of a trilayer stamp. ( b ) A microscope image and ( c ) surface profile of the stamp monitored by a phase measurement with an interface microscope. The stamp surface has a high flatness because of the flatness of the glass plate. Full size image Substrate treatment We used an n -doped silicon plate with a 300-nm-thick thermally grown SiO 2 layer as the substrate. After being cleaned, the surface was treated with 1,1,1,3,3,3-hexamethyldisilazane, trichloro(octyl)silane (OTS-8), OTS-18, FAS-17 or FOTS-8. All the obtained substrates have highly hydrophobic surfaces with high water (or TCB) contact angles of 92° (52°), 106° (50°), 110° (57°), 110° (70°) and 111° (74°) for the HMDS-, OTS-18-, OTS-8-, FAS-17- and FOTS-8-treated surfaces, respectively. Preparation of semiconductor solution We purchased the P3HT (Merck Co., Ltd), PQT-12 (American Dye Source, Inc.) and PBTTT (Merck Co., Ltd.). The commercially available P3HT was purified through Soxhlet extraction with hexane and dichloromethane [29] , to afford the product with a molecular mass ( M ) of 71 kDa, a polydispersity index (PDI) of 1.67 and a regio regularity of 96%. The PQT-12 ( M =33 kDa and PDI=2.9) and PBTTT ( M =38 kDa and PDI=1.98) were used without further purification. The semiconductors were dissolved in TCB at 65 °C for 30 min and then filtered through a 0.45-μm pore size poly(tetrafluoroethylene) membrane filter. We used 0.1 wt% semiconductor solution in anhydrous TCB for the push coating and 0.4 or 0.6 wt% solution for the spin coating. Preparation of spin-coated films In contrast to the push coating, it was quite difficult to fabricate films by spin coating when the high b.p. solvent, such as TCB, and highly hydrophobic surfaces were used. This is because most of the solution is lost during the initial spinning process before the films are grown. A former report was restricted to the use of only toluene (b.p. 110.6 °C); the toluene has lower surface tension than other solvents [10] . We fabricated spin-coated films using 0.4 wt% P3HT solution in TCB on hydrophilic and hydrophobic surfaces, the appearance of which is shown in Supplementary Fig. S1 . The film coverage is almost 50% on the hydrophilic surface and less than a few per cent on the hydrophobic surface. To increase the coverage, we used a smaller-area substrate with specific surface treatments; the perimeter of the area is converted into a hydrophilic surface using ultraviolet irradiation with excimer lamp, which suppresses the loss of solution during the initial spinning process. The coverage improves to around 50% on hydrophobic surface, although the film is not uniform. X-ray diffraction The synchrotron-radiated X-ray measurements were conducted at the BL-8B line of the KEK (High Energy Accelerator Research Organization) Photon Factory. The X-rays that we used had an energy of 18 keV (wavelength 0.6885 Å). The monochromated beam was focused at the sample position with beam size of 300 × 300 μm 2 . The Bragg reflections were detected by a cylindrical imaging-plate diffractometer (SPD; Rigaku, Tokyo), where the oscillation photographs were taken at Δ θ =5° and |2 θ |<20°. Device fabrication To fabricate the bottom-contact, bottom-gate TFTs, source and drain electrodes (Au 30 nm/Cr 5 nm) were first prepared by a photolithographic technique before the semiconductor film growth. We used five channel lengths, 5, 10, 20, 50 and 100 μm, and a channel width of 5 mm. The device characteristics were measured using a semiconductor parametric analyser (E5270A; Agilent). How to cite this article: Ikawa, M. et al. Simple push coating of polymer thin-film transistors. Nat. Commun. 3:1176 doi: 10.1038/ncomms2190 (2012).